The endoskeletal origin of the turtle carapace The turtle body plan, with its solid shell, deviates radically from those of other tetrapods. The dorsal part of the turtle shell, or the carapace, consists mainly of costal and neural bony plates, which are continuous with the underlying thoracic ribs and vertebrae, respectively. Because of their superficial position, the evolutionary origins of these costo-neural elements have long remained elusive. Here we show, through comparative morphological and embryological analyses, that the major part of the carapace is derived purely from endoskeletal ribs. We examine turtle embryos and find that the costal and neural plates develop not within the dermis, but within deeper connective tissue where the rib and intercostal muscle anlagen develop. We also examine the fossils of an outgroup of turtles to confirm that the structure equivalent to the turtle carapace developed independently of the true osteoderm. Our results highlight the hitherto unravelled evolutionary course of the turtle shell. Two types of skeletal systems are recognized in vertebrates, the exoskeleton composed of the dermal bones and the cartilaginously preformed endoskeleton [1] , [2] , [3] . For the past 200 years, the origin of the turtle carapace has remained unclear, and several different hypotheses about incorporation of the exoskeletal components into the costal and neural plates ( Fig. 1 , Supplementary Fig. S1 ) have been proposed [4] , [5] , [6] , [7] , [8] , [9] , [10] , [11] , [12] , [13] , [14] , [15] , [16] , [17] , [18] , [19] , [20] , although the exoskeletal origin of the accessory bones that surround the costo-neural plates marginally, namely the nuchal, peripheral, suprapygal and pygal plates, is widely accepted. One hypothesis assumes that costo-neural elements contain both the endo- and exoskeletal materials—in particular, dermal elements called the osteoderm [5] , [8] , [13] , [14] , [15] , [18] , [19] . For shell acquisition, the osteoderms of the ancestral animal was thus thought to have fused with the axial skeletal elements (ribs and vertebrae) underneath. Osteoderms are also seen in other tetrapods (for example, crocodilians and armadillos) [3] , [21] , [22] , [23] , and the most conspicuous examples are found in extinct animals, namely the mammalian glyptodontids, in which exoskeletal elements form a thoracic shell. However, in contrast to the completely immovable shell seen in the turtle, the shells of the above-mentioned armoured tetrapods are not linked directly to the vertebral column or the rib cage, allowing free movement of the rib cage with the surrounding intercostal muscles. 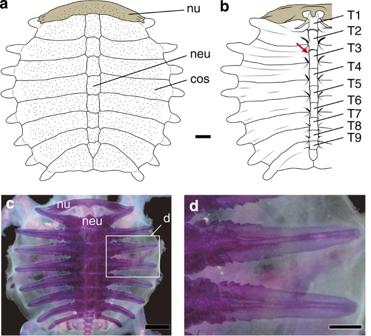Figure 1: Carapace of Chinese soft-shelled turtlePelodiscus sinensis. (a) Dorsal view. Scale bar, 1 cm. (b) Right half in ventral view. Red arrow indicates the costovertebral articulation. (c) Cleared and double-stained juvenile specimen. Scale bar, 5 mm. (d) Enlarged image of the immature costal plates inc. Box incindicates the position ofd. Scale bar, 2 mm. cos, costal plate; T1–T9, thoracic vertebra numbers; neu, neural plate; nu, nuchal. Figure 1: Carapace of Chinese soft-shelled turtle Pelodiscus sinensis . ( a ) Dorsal view. Scale bar, 1 cm. ( b ) Right half in ventral view. Red arrow indicates the costovertebral articulation. ( c ) Cleared and double-stained juvenile specimen. Scale bar, 5 mm. ( d ) Enlarged image of the immature costal plates in c . Box in c indicates the position of d . Scale bar, 2 mm. cos, costal plate; T1–T9, thoracic vertebra numbers; neu, neural plate; nu, nuchal. Full size image The second hypothesis assumes the endoskeletal origin of the costo-neural carapace, maintaining that the costal and neural plates were simply acquired by modification of the axial skeleton and, therefore, that the major parts of the carapace were formed solely from the endoskeleton [4] , [7] , [11] . Lastly, in the third hypothesis, superficially translocated endoskeletal elements were thought to induce heterotopically exoskeletal osteogenesis of the carapace. Recent observations of the embryonic turtle suggest that heterotopic shifts of the ribs occur during development: rib primordia translocated into the dermis induce membranous ossification to differentiate flanges on the craniocaudal aspects of the rib shafts and thus complete the costal plate. The superficial shift of the ribs, initially arising endochondrally, is thought to cause a new tissue interaction in the new location (that is, the dermis) [16] , [17] . Here through a comparative developmental analysis, we demonstrate that the costal and neural plates are assigned to be hypertrophied ribs and vertebrae, respectively. These results indicate that the major part of the turtle carapace evolved solely by modification of the endoskeleton (that is, second hypothesis). Furthermore, in the fossil record, we recognized that precursors of carapace in some non-turtle diapsid reptiles developed also as an endoskeleton. The ribs of these reptiles are not only expanded in shape, as seen for examples, in extant anteaters [24] or a Permian reptile Eunotosaurus [25] , but also laterally (nearly horizontally) projected as in the turtles. The genetic basis relevant to the carapace evolution is, therefore, likely to have deeper history than the split of the turtle lineage. The embryonic development of costal plates We observed the embryonic histology of the Chinese soft-shelled turtle ( Pelodiscus sinensis ) to elucidate the embryonic environment of the developing costo-neural plates, which has long been ambiguous [5] , [6] , [7] , [10] , [11] , [12] , [16] , [18] . We found that the development of the costo-neural plates proceeds within the connective tissue associated with the axial muscles, under the dermis ( Fig. 2 ). Specifically, at stage 17, the intercostal muscles are found between ribs: these tissues are embedded in thin connective tissue ( Fig. 2a ). At stage 18, the dermis appears as mesenchyme with a matrix that is stained with Alcian-blue; it has a clear boundary with the underlying subdermal connective tissue and the ribs ( Fig. 2b ). At this stage, the intercostal muscles begin to degenerate, but the subdermal layer remains at subsequent stages especially near the ribs ( Fig. 2b ). Thus the ribs remain to be encapsulated in the subdermal cell mass ( Fig. 2c , sdc) under the dermis at stage 21 and thereafter. In the following stages ( Fig. 2d ), the rib periosteum expands craniocaudally within the subdermal cell mass. The intercostal muscles disappear, but the subdermal layer remains present ( Fig. 2d , sdc). In the rib periosteum of stage 27 embryos, the flanges of the costal plates appear as membranously ossified bony trabeculae extending from the craniocaudal aspects of the bone collar of the ribs ( Fig. 2e , btr). In the post-hatching development, these trabeculae extend farther outward from the rib shaft to complete the costal plate ( Supplementary Fig. S2 ). The neural plate expands along the surface of the intrinsic back muscles, outside of the dermis ( Supplementary Fig. S3 ). 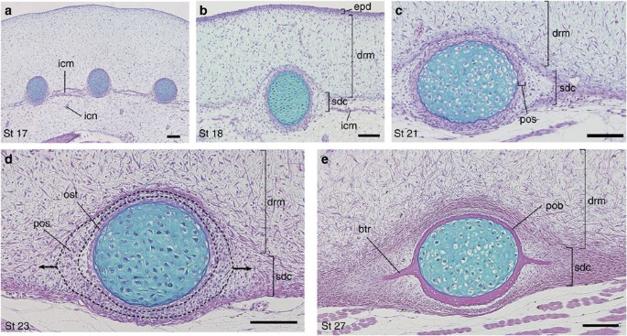Figure 2: Development of the costal plate in the turtle. Hematoxylin-eosin-Alcian-blue-stained cross-sections of the ribs of the Chinese soft-shelled turtle (Pelodiscus sinensis). (a) Stage 17. Scale bar, 100 μm. (b) Stage 18. Scale bar, 100 μm. (c) Stage 21. Scale bar, 100 μm. (d) Stage 23. Scale bar, 100 μm. Arrows indicate direction of expansion of the periosteum (pos). (e) Stage 27. Scale bar, 100 μm. btr, bony trabecula; drm, dermis; epd, epidermis; icm, intercostal muscle; icn, intercostal nerve; ost, osteoblast; pob, periosteal bone collar; pos, periosteum; sdc, subdermal connective tissue. Figure 2: Development of the costal plate in the turtle. Hematoxylin-eosin-Alcian-blue-stained cross-sections of the ribs of the Chinese soft-shelled turtle ( Pelodiscus sinensis ). ( a ) Stage 17. Scale bar, 100 μm. ( b ) Stage 18. Scale bar, 100 μm. ( c ) Stage 21. Scale bar, 100 μm. ( d ) Stage 23. Scale bar, 100 μm. Arrows indicate direction of expansion of the periosteum (pos). ( e ) Stage 27. Scale bar, 100 μm. btr, bony trabecula; drm, dermis; epd, epidermis; icm, intercostal muscle; icn, intercostal nerve; ost, osteoblast; pob, periosteal bone collar; pos, periosteum; sdc, subdermal connective tissue. Full size image We also found that the outward growth of bony trabeculae with an expansion of the periosteum ( Fig. 2d ) is not a turtle-specific developmental pattern, but is comparable to rib development in the chicken ( Fig. 3 ). In the stage 40 chicken embryo, as in P. sinensis at stage 23 and thereafter, the rib periosteum expands to form bony trabeculae that extend outward from the periosteal bone collars at the insertions of the intercostal muscles. Taken together, the initial development of the turtle’s costal plate and morphogenesis of the avian rib follow the comparable sequence, and that the costal plate can be identified as a morphologically modified rib. The morphological difference between the costal plate and the avian rib is attributable to differences in the magnitude of outward growth of the bony trabeculae. Outward growth of the trabeculae in turtles is so extensive that the rib invades the intercostal space as the costal plate. 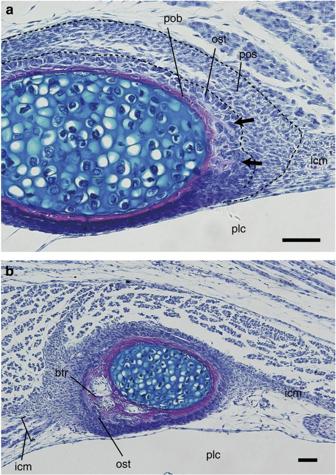Figure 3: Membranous bone formation of the rib in birds. Hematoxylin-eosin-Alcian-blue-stained cross-section of the rib in a chicken (Gallus gallus) embryo at stage 40. (a) Delicate bony trabeculae (osteoids) at the insertion of the intercostal muscle (icm). Arrows indicate protrusion of bony trabeculae. Scale bar, 100 μm. (b) Bony trabeculae at the insertion of the intercostal muscle (icm). Scale bar, 100 μm. btr, bony trabecula; plc, pleural cavity; pob, periosteal bone collar; pos, periosteum; ost, osteoblast. Figure 3: Membranous bone formation of the rib in birds. Hematoxylin-eosin-Alcian-blue-stained cross-section of the rib in a chicken ( Gallus gallus ) embryo at stage 40. ( a ) Delicate bony trabeculae (osteoids) at the insertion of the intercostal muscle (icm). Arrows indicate protrusion of bony trabeculae. Scale bar, 100 μm. ( b ) Bony trabeculae at the insertion of the intercostal muscle (icm). Scale bar, 100 μm. btr, bony trabecula; plc, pleural cavity; pob, periosteal bone collar; pos, periosteum; ost, osteoblast. Full size image Additional support for the axial skeletal identity of the costo-neural plates is derived from comparison with the osteoderms. In the American alligator ( Alligator mississippiensis ), the osteoderm develops within the dermis in close association with the epidermis, implying the involvement of the epithelial–mesenchymal interactions in its development [21] ( Supplementary Fig. S4 ). Thus, the mechanism of development of the osteoderm is quite different from that of the costo-neural plates. Collectively, our comparative analyses of these embryonic developments suggest that the turtle’s costo-neural plates are entirely of endoskeletal origin (that is, the second hypothesis). Turtle-type carapaces of some basal diapsids The results of our embryonic analyses explain the nature of the stem turtle [26] Odontochelys semitestacea , in which the carapace does not form a closed-shell structure. The rib shaft of Odontochelys has craniocaudal plate-like extensions from the rib shaft ( Supplementary Fig. S5 ). This is best explained by the reasoning that Odontochelys was endowed with the same developmental background of the costal plate as observed in other turtles. The articulation between the rib and the vertebra in Odontochelys is immovable (nearly synarthrosis condition; Supplementary Fig. S5 ), indicating that this animal already had a rigid shell instead of an intercostal muscle system. Furthermore, we found examples in the fossil record to corroborate the evolutionary course from axial endoskeleton to the turtle-type rigid shell. Recently reported specimens of the Middle Triassic marine reptile Sinosaurosphargis yunguiensis [27] , for example, possess laterally extended plate-like ribs and overlying osteoderms ( Fig. 4 ; Supplementary Fig. S6 ). Similar skeletal configuration has been reported in the basal sauropterygian Henodus chelyops [28] . 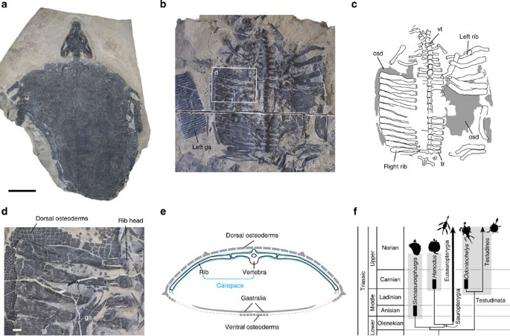Figure 4: Middle Triassic marine reptileSinosaurosphargis yunguiensis. (a) Dorsal view of the holotype, IVPP V17040, preserving the skull and skeleton of the trunk region. Scale bar for the upper panels (a–c), 10 cm. (b) Ventral view of the paratype, IVPP V16076, preserving the skeleton of the trunk region. (c) Line drawing ofb. (d) Enlarged image of the ribs and vertebrae inb. Box inbindicates the position ofd. Scale bar, 1 cm. (e) Schematic structure of a transverse section of the rib cage inS. yunguiensis. (f) Phylogeny of the taxa examined. osd, osteoderm; ga, gastralia; tr, transverse process; vt, vertebra. Figure 4: Middle Triassic marine reptile Sinosaurosphargis yunguiensis . ( a ) Dorsal view of the holotype, IVPP V17040, preserving the skull and skeleton of the trunk region. Scale bar for the upper panels ( a – c ), 10 cm. ( b ) Ventral view of the paratype, IVPP V16076, preserving the skeleton of the trunk region. ( c ) Line drawing of b . ( d ) Enlarged image of the ribs and vertebrae in b . Box in b indicates the position of d . Scale bar, 1 cm. ( e ) Schematic structure of a transverse section of the rib cage in S. yunguiensis . ( f ) Phylogeny of the taxa examined. osd, osteoderm; ga, gastralia; tr, transverse process; vt, vertebra. Full size image Sinosaurosphargis possesses a flat articular facet for the rib on each vertebral transverse process, indicating restriction of rib movements ( Fig. 4d ). The rib bears plate-like extensions both craniad and caudad from the shaft. These extensions are so extensive that there is only a small amount of space between neighbouring ribs along almost the entire length of their edges. This rib morphology, along with the limited movability, implies that the intercostal muscles have been reduced, being replaced by the plate-like ribs. This morphology is highly reminiscent of the ribs of turtles and Odontochelys . In addition, the neural spine is low rather than high, and thus the epaxial muscles may have been only poorly developed. Because of the reduction of the intercostal and epaxial muscles, the plate-like ribs of Sinosaurosphargis were likely embedded superficially in the dorsal aspect of the body wall. These lines of anatomical similarity indicate that the plate-like rib of Sinosaurosphargis and the costal plate of the turtle reflect the equivalent developmental processes, in which the immovable shells grow within the subdermal connective tissue normally occupied by the intercostal muscle layer. The ribs of Sinosaurosphargis are overlain by a pavement of rectangular skeletal plates ( Fig. 4e ; Supplementary Fig. S6 ). The outer surfaces of these rectangular plates are ornamented by keels or rugosities, whereas the inner surfaces are poorly ornamented, evidencing a characteristic feature of the osteoderm, namely an intimate interaction with the integument. Recent molecular-based phylogenetic analyses of living taxa have corroborated the affinity of the turtles to archosaurs [29] , [30] , [31] , [32] , [33] . Notably, a genome-wide molecular-based phylogenetic analysis demonstrated that the turtles are related closer to archosaurs than to lepidosaurs and nested in the diapsid clade [34] . Recent comprehensive morphology-based phylogenetic analyses of amniotes also showed that turtles belong to diapsids [35] , [36] . As to interrelationships among diapsids, analyses with denser taxon sampling have recently demonstrated that the turtles and sauropterygians are likely settled in an identical clade, which is related either more closely to lepidosaurs [37] , [38] or more closely to archosaurs [39] , [40] . In addition, a phylogenetic analysis on Sinosaurosphargis has placed this taxon in the sister group of sauropterygians, together with thalattosaurs [27] . Therefore, although there still remain debates as to the positions of these taxa within diapsids [41] , [42] , it is reasonable that the turtles, the sauropterygians, and Sinosaurosphargis are settled in an identical clade ( Fig. 4f ), in the light of most of the current hypotheses [27] , [35] , [38] , [39] , [40] . Recent detailed studies on embryonic development [17] , [18] and bone histology [18] , [43] have repeatedly assumed possibilities that exoskeletal components contribute to the costal plate. However, the data about the costal plate development in this study favour the purely endoskeletal origin of the costal plate. It is reasonable that the expansion of the periosteum has a crucial role in the development of costal plates in all the turtles. Importantly, the classification of ossification and that of the skeletal system are fundamentally different. Although the exoskeletal, dermal elements are generated purely through membranous ossification, this process should be regarded primarily as a histogenetic mode of ossification, and does not decisively correlate with exoskeleton as a skeletal system [1] , [2] , [44] . This is because membranous ossification is also associated with the endochondrally preformed endoskeletal elements, as is typically seen in the late phase of development of the shafts of long bones. The latter are membranous bones, not dermal. Moreover, reliable molecular markers for identifying dermal bones have not been reported so far: the cranial dermal bone is molecularly distinguishable only in a transient coexpression of both osteogenic and chondrogenic markers [45] , and developmental regulations of postcranial dermal bones, or osteoderms, are unknown. Therefore, embryonic environments of developing bones, rather than histogenesis or gene expressions, are the key to the discrimination between endo- and exoskeletons. In the previous study on the embryonic development of a different species of turtle ( Trachemys scripta ), a secretion of the bone morphogenetic protein (BMP) signalling from the rib was observed, and a hypothesis on the molecular profile, in which the BMP signalling induce the dermal cells to be differentiated into osteoblasts to complete the costal plate, has been proposed (third hypothesis) [17] . This hypothesis is, however, not consistent with the mode of heterotopic ossification in the dermis as was observed in an experiment of heterotopic periosteal cell grafting [46] . When the periosteal cells were grafted to the dermis in rabbits, the BMP signalling expressed around the grafted periosteal cells as in the turtle ribs, but the osteoblasts, which produce heterotopic bones in the dermis, were all derived from the grafted periosteal cells. Recent analyses showed that, in the development of long bones, the perichondrial cells migrate internally to be differentiated into osteoblasts to produce bone trabeculae [47] . Based on these capabilities of periosteal/perichondrial cells, along with our observations, it is more parsimonious that the periosteal cells of the ribs generate the costal plates throughout the development, than that the osteoblasts are differentiated from the dermal cells by induction secreted from the ribs, although the periosteum is dismantled to lose its clear structure in the later developmental stage (in the case of P. sinensis , post-hatching development; Supplementary Fig. S2 ). On the other hand, bone histology of costal plates indicates the influence of the dermis upon outer layers of costal plates, in particular in later phase of the development [18] , [43] , where collagen fibre bundles are incorporated through metaplastic bone formation [48] . These evidences do not contradict the endoskeletal nature of costal plates, because the dermis often affects outer layers of superficially exposed parts of bones, for examples, the distal part of the distal phalanx ( Supplementary Fig. S7 ). Furthermore, above presented fossil evidences imply how ribs were evolved into solid shells. The axial musculoskeletal system of the stem turtle Odontochelys represents an early stage of carapace evolution, thus the origin of the rigid carapace structure preceded the encapsulation of the scapular blade into the carapace in the turtle evolution [49] . The turtle-type carapace can be seen in other diapsids outside of the turtle clade, namely in Sinosaurosphargis and in Henodus . According to recent phylogenetic analyses, these reptiles are most likely to represent outgroup taxa closer to the turtle than are any living reptiles ( Fig. 4f ), although they have not undergone some of the morphological changes observed in the turtle, such as internal positioning of the scapula. Our reconstruction of rib cage anatomy of Sinosaurosphargis underlines the similarity with the turtle carapace. The ribs of Sinosaurosphargis are not only plate-like in shape, but also laterally projected as in the turtles ( Fig. 4e ), rather than curved ventrally as in most amniotes, implying that the rib cage of Sinosaurosphargis exclusively functioned as a shell. In some sauropterygians, the ribs are also projected laterally in the dorsal aspect of the trunk, and the pectoral girdle is laid in the ventral position relative to the rib cage [50] , [51] . This unusual construction seen in their trunk skeleton is reminiscent of the rib patterning of the turtles [16] , [49] , [52] , [53] , [54] . Taking this into account, it seems reasonable to hypothesize that a shared genetic basis for rib patterning was evolved in a more inclusive clade than the turtles, and along with the hypertrophy of ribs, yielded the endoskeletal shell structures in Sinosaurosphargis , in Henodus, and in the turtles ( Fig. 5 ). The recurrent, or discontinuous distribution of the endoskeletal shell structure in phylogeny does not necessarily exclude the possibility of a shared ancestry of the genetic basis (cf. Hall [55] ). 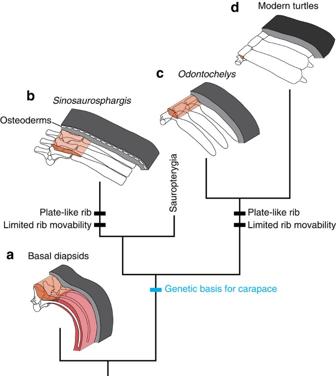Figure 5: Evolution of the carapace by modification of the rib. (a) Basal diapsids, possessing the movable rib cage. (b)Sinosaurosphargis(Middle Triassic). The laterally projected ribs were expanded to form the carapace, and the intercostal muscles were likely poorly developed. (c) Basal turtle species,Odontochelys(Late Triassic). The laterally projected ribs were expanded to form the carapace, and the intercostal muscles were likely poorly developed. (d) Modern turtles. The intercostal muscle anlage degenerates during embryonic development. Grey, integument; orange, epaxial muscles; red, hypaxial muscles including intercostal muscles. Figure 5: Evolution of the carapace by modification of the rib. ( a ) Basal diapsids, possessing the movable rib cage. ( b ) Sinosaurosphargis (Middle Triassic). The laterally projected ribs were expanded to form the carapace, and the intercostal muscles were likely poorly developed. ( c ) Basal turtle species, Odontochelys (Late Triassic). The laterally projected ribs were expanded to form the carapace, and the intercostal muscles were likely poorly developed. ( d ) Modern turtles. The intercostal muscle anlage degenerates during embryonic development. Grey, integument; orange, epaxial muscles; red, hypaxial muscles including intercostal muscles. Full size image Significantly, it is informative for the carapace evolution that Sinosaurosphargis possess osteoderms. By the criterion of conjunction for homology [56] , the possibility that the plate-like rib of Sinosaurosphargis includes exoskeletal derivatives is rejected, matching the prediction that the superficially positioned turtle-type carapace evolved independently of the exoskeleton ( Fig. 5 ). Our study reveals the historical continuity between the axial endoskeleton and the turtle carapace, bridging the gap in body plan between the turtle and other tetrapods ( Fig. 5 ). The exoskeleton, which often forms a bony protection in vertebrate evolution, was not the main contributor to the evolution of the turtle carapace. Rather, the costo-neural plates of the turtle carapace solely represent different character states [57] of the rib and vertebra, respectively. Our findings further imply that the genetic basis for the establishment of the turtle carapace, at least partly dates back to a more inclusive and basal phylogenetic level than the origin of the turtle. Embryonic histology Chinese soft-shelled turtle ( Pelodiscus sinensis ) eggs were purchased from a local farm in Japan and incubated at 30 °C. The embryos were staged according to the Tokita and Kuratani stage table [58] and fixed with Bouin’s fixative. Chicken ( Gallus gallus ) eggs were purchased from a local farm in Japan and incubated at 38 °C under moist conditions. The embryos were staged according to the Hamburger and Hamilton stage table [59] and fixed with Serra’s fixative. Histological sections of the turtles (6 μm) and the chickens (8 μm) were stained with Alcian-blue, hematoxylin and eosin. Eggs of the American alligator ( Alligator mississippiensis ) were collected legally from the Rockefeller Wildlife Refuge, Cameron, Louisiana. The embryos were staged according to the Ferguson stage table [60] and fixed with Serra’s fixative. Histological sections of the alligators (8 μm) were stained with Alcian-blue, hematoxylin and eosin, and were also stained immunohistochemically (anti-acetylated tubulin antibody, T6793, Sigma-Aldrich, St Louis, Missouri, USA, at a dilution of 1:400). The samples were transported with the permission of CITES (Certificate No. 11US37892A/9). Fossils Anatomical data for Odontochelys semitestacea [26] (IVPP V 15653) from the Upper Triassic Falang Formation, Guizhou Province, China, and for Sinosaurosphargis yunguiensis [27] (IVPP V 17040 and V 16076) from the Middle Triassic Guanling Formation, Yunnan Province, China, were collected for this study. These specimens are housed at the IVPP (Institute of Vertebrate Paleontology and Paleoanthropology), Beijing, China. How to cite this article: Hirasawa, T. et al. The endoskeletal origin of the turtle carapace. Nat. Commun. 4:2107 doi: 10.1038/ncomms3107 (2013).